Gold-catalyzed stereoselective cycloisomerization of allenoic acids for two types of common natural γ-butyrolactones γ-( E )-Vinylic and γ-alkylic γ-butyrolactones are two different types of lactones existing extensively in animals and plants and many of them show interesting biological activities. Nature makes alkylic γ-butyrolactones by many different enzymatic lactonization processes. Scientists have been mimicking the natural strategy by developing new catalysts. However, direct and efficient access to γ-( E )-vinylic γ-butyrolactones is still extremely limited. Here, we wish to present our modular allene approach, which provides an efficient asymmetric approach to ( E )-vinylic γ-butyrolactones from allenoic acids by identifying a new gold complex as the catalyst. Based on this cycloisomerization strategy, the first syntheses of racemic xestospongiene and xestospongienes E, F, G, and H have been realized and the absolute configurations of the chiral centers in xestospongienes E and F have been revised. In addition, by applying a C–O bond cleavage-free hydrogenation, the syntheses of naturally occurring γ-alkylic γ-lactones, ( R )-4-tetradecalactone, ( S )-4-tetradecalactone, ( R )-γ-palmitolactone, and ( R )-4-decalactone, have also been achieved. Natural products are a big treasure for human beings, which exhibit rich academic and industrial potentials due to their structural diversity and biological activities. As we know, γ-butyrolactones with common structures of γ-( E )-vinylic and alkylic γ-butyrolactones, E- I [1] , [2] , [3] , [4] and II [5] , [6] , [7] , [8] , [9] , [10] , exist extensively in nature and many of them have been identified with interesting biological potentials, such as anti-HIV [1] , anti-fungal [2] , [9] , cytotoxic [3] , anti-bacterial [7] , anti-proliferative [8] activities, etc., featuring applications in pharmacy (Fig. 1 ). Some of these lactones, especially for aliphatic γ-butyrolactones, are also common flavor source in plants and food, which involved in several metabolic pathways [11] . Fig. 1 Representative examples of γ-( E )-vinylic and γ-alkylic-γ-butyrolactones. a Common structure unit and representative examples of γ-( E )-vinylic γ-butyrolactones ( E- I ); b Common structure unit and representative examples of γ-alkylic γ-butyrolactones ( II ) Full size image So far, very few highly selective asymmetric synthesis of E- I -type γ-butyrolactones with a trans 1,3-disubstituted C=C bond has been reported [12] , [13] . The approaches for the synthesis of unique γ-(2,2-disubstituted or 1-iodo) vinylic γ-butyrolactones [14] , [15] , [16] , [17] , [18] are not applicable for the synthesis of the natural γ-butyrolactones due to the substrate limitation. It is well reasoned that in the Au-catalyzed enantioseletcive approach the control of E / Z selectivity and enantioselectivity are most likely the challenge when 6-mono-substituted allenoic acids were used (Fig. 2d ) [14] , [15] , [16] . We envisioned a Au-catalyzed cycloisomerization [19] , [20] , [21] , [22] , [23] , [24] , [25] of optically active 4,5-alkadienoic acids, readily available from terminal alkynes and aldehydes, for the direct access to various natural and non-natural enantioenriched E- I -type common γ-butyrolactones, which could further be easily hydrogenated to provide naturally occurring γ-alkylic γ-butyrolactones II (Fig. 2e ). The latter was usually prepared via the lactonization (Fig. 2a ) [26] , [27] , [28] , [29] , Baeyer-Villiger oxidation (Fig. 2b ) [30] , and dihydroxylation-lactonization-elimination (Fig. 2c ), etc [31] , [32] , [33] , [34] . The challenge for strategy in Fig. 2e is the efficiency of axial-to-central chirality transfer [35] , [36] , [37] , [38] , [39] , [40] , [41] , [42] , [43] and the control of Z / E selectivity ( E - I vs. Z - I , which after hydrogenation would afford the enantiomers of lactones II , respectively, thus, leading to a much lower ee) during the cyclic anti-nucleometalation and the efficiency of the proto demetalation process to deliver the required 1,3-disubstituted E -C=C bond finishing the catalytic cycle. Overall it is highly desirable to identify a suitable ligand L for a much more stable complex I over complex II . Fig. 2 Known approaches and the designed general protocol to γ-butyrolactones E - I and II . a Nature’s enzymatic approaches; b Baeyer–Villiger oxidation; c Alkenoate dihydroxylation; d Allene enantioselective approach described in refs. [14] , [15] , [16] . e Au-catalyzed chirality transfer-based asymmetric cyclization of allenoic acids (this work) Full size image Herein, we present the highly stereoselective cycloisomerization of optically active 5-monosubstituted 4,5-alkadienoic acids affording various non-natural and natural enantioenriched γ-( E )-alkenyl-γ-butyrolactones by using AuCl(LB-Phos) as the catalyst. Synthesis of AuCl(LB-Phos) At the beginning, we treated ( R a )-4,5-tridecadienoic acid ( R a )- 5a (for its synthesis from aldehyde and terminal alkyne, see: Supplementary Tables 1 and 2 ) as the model substrate. 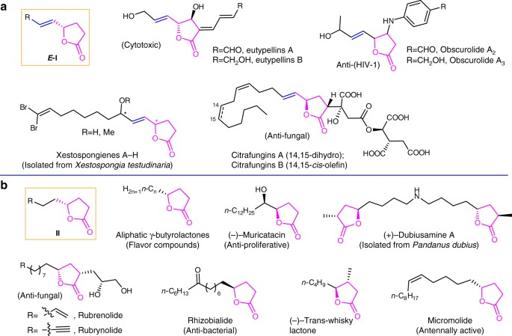Fig. 1 Representative examples of γ-(E)-vinylic and γ-alkylic-γ-butyrolactones.aCommon structure unit and representative examples of γ-(E)-vinylic γ-butyrolactones (E-I);bCommon structure unit and representative examples of γ-alkylic γ-butyrolactones (II) After screening of some commonly used gold catalysts such as AuCl, AuCl(IPr), Au 2 Cl 2 (dppm), Au 2 Cl 2 (dppm) combined with AgOTs was identified as the first generation catalyst to afford the desired γ-1 (E) - alkenyl ( S )-γ-butyrolactone ( S , E )- 6a in a quantitative yield with a E / Z selectivity of 93:7 and 96% ee in CHCl 3 at room temperature for 3 h (Table 1 , entry 1). For the purpose of improving the E/Z selectivity, we tried to identify a more stereoselective catalyst. Based on our recent development of monophosphine ligands [44] , some of the gold complexes of these ligands have been prepared. AuCl(LB-Phos), the structure of which was determined by X-ray single crystal diffraction study (Fig. 3 ) [45] , is one of them. Fig. 3 Complex AuCl(LB-Phos). Synthesis and ORTEP representation of AuCl(LB-Phos) Full size image Optimization of reaction conditions With this rather sterically bulky AuCl(LB-Phos), gladly, an E / Z selectivity of 97:3 with 100% yield and 97% ee was observed, indicating that the new catalyst was able to control both the C=C stereoselectivity and ensure the efficiency of chirality transfer (Table 1 , entry 2). Inspired by this result, we explored the effect of solvents: CH 2 Cl 2 gave a similar E / Z and ee (Table 1 , entry 3), while 1,2-DCE led to a rather poor E / Z selectivity of 91:9 (Table 1 , entry 4); CH 3 NO 2 showed a better E -selectivity of 98:2, but a much lower ee of 90% (Table 1 , entry 6); other solvents such as toluene, dioxane, and CH 3 CN failed to yield any better results even with a prolonged time of 12 h (Table 1 , entries 5, 7–8). In the absence of AgOTs, the expected product 6a was obtained in only 8% yield with 92% recovery of ( R a )- 5a after 24 h (Table 1 , entry 9), and the lactonization couldn’t take place by just using AgOTs (Table 1 , entry 10), indicating the significance of the gold-catalysis. Examining the effect of different salts showed the importance of the counter anion: AgPF 6 resulted in the same E/Z -selectivity but with a lower ee of 92% (Table 1 , entry 11), while other common silver salts such as AgOTf, AgSbF 6 , and AgOAc, etc. all caused a dropped E / Z selectivity ranging from 82:18 to 93:7 (Table 1 , entries 12–16). Thus, we defined the standard reaction conditions as follows: 5 mol% Au(LB-Phos)Cl/AgOTs in CHCl 3 at 25 °C for 3 h (Table 1 , entry 2). 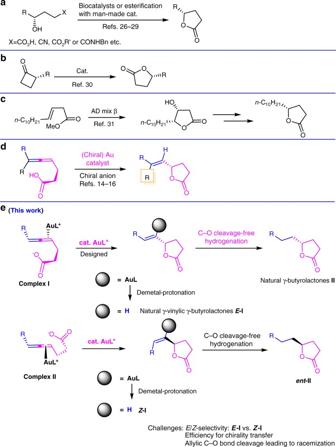Fig. 2 Known approaches and the designed general protocol to γ-butyrolactonesE-IandII.aNature’s enzymatic approaches;bBaeyer–Villiger oxidation;cAlkenoate dihydroxylation;dAllene enantioselective approach described in refs.14,15,16.eAu-catalyzed chirality transfer-based asymmetric cyclization of allenoic acids (this work) Table 1 Optimization of the reaction conditions for AuCl(LB-Phos)-catalyzed stereoselective cyclization of 4,5-allenoic acid ( R a )- 5a Full size table Substrate scope With the optimized reaction conditions in hand, differently substituted 4,5-allenoic acids ( R a )- 5 were treated with AuCl(LB-Phos) to afford γ-1 (E) - alkenyl ( S )-γ-butyrolactones in high yields (93–98%) with an excellent axial-to-center chirality transfer and E / Z -selectivity (up to >99:1 E / Z ) (Table 2 ): R could be primary alkyl: n -heptyl ( 6a ), n -butyl ( 6b ), n -undecyl ( 6c ), and phenylethyl ( 6g ), or branched alkyl: i -Pr ( 6d ), and Cy ( 6e ). The reaction of benzyl-substituted ( R a )- 5f should be conducted at −40 °C for 6 h to keep the enantioselectivity due to the observed racemization at 25 °C ( 6f ) (compare entry 6 with entry 7 in Table 2 ). Functional groups including benzyl group, C=C, and C≡C bonds were also tolerated ( 6f , 6g , 6h , and 6i ). Table 2 Highly stereoselective synthesis of ( S , E )- 6 Full size table As expected, the enantiomer ( R , E )-butyrolactone ( 6j ) could also be prepared from the enantiomer of the starting allene, ( S a )-4,5-dienoic acid ( S a )- 5j , in a high yield and an excellent E / Z -selectivity (Fig. 4a ). 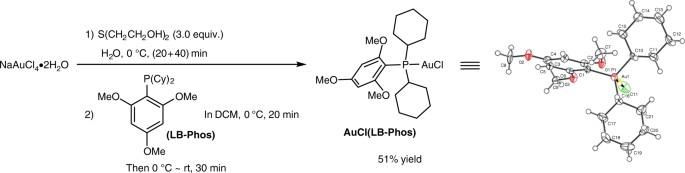Fig. 3 Complex AuCl(LB-Phos). Synthesis and ORTEP representation of AuCl(LB-Phos) After some further optimization (see Supplementary Table 3 ), a 10 mmol scale reaction with just 1.5 mol% each of AuCl(LB-Phos) and AgOTs in CHCl 3 at −20 °C for 15 h was realized, delivering an excellent yield of chiral lactone ( S , E )- 6b with 97% ee and 98:2 E / Z selectivity (Fig. 4b ). Fig. 4 Extended scope of Au-catalyzed cycloisomerization reaction. a Synthesis of the enantiomer ( R , E )-butyrolactone 6j ; b Gram scale synthesis for γ-butyrolactone ( S , E )- 6b Full size image The effect of different gold catalysts The results of different gold catalysts combined with AgOTs in CHCl 3 are listed in Table 3 , which showed that AuCl(LB-Phos) was indeed the best catalyst (Table 3 , entry 6). Table 3 The effect of different gold catalyst on the stereoselective cyclization of 4,5-allenoic acid ( S a )- 5m Full size table Synthesis of racemic xestospongiene Such a strategy should deliver a direct entry to the optically active natural γ-butyrolactone with common structure E - I as shown in Fig. 1a . Xestospongienes are a series of brominated polyunsaturated lipids isolated from the Chinese marine sponge Xestospongia testudinaria (shown in Fig. 1a ) [4] . No total synthesis has been reported yet. Thus, 7-(( tert -butyldimethylsilyl)oxy)heptanal 7 underwent 1,2-addition reaction with ethyl magnesium bromide to yield propargylic alcohol 8 . Methylation of 8 via deprotonation with NaH, followed by quenching with MeI, and subsequent removal of the TBS group via acidic hydrolysis yielded the primary alcohol 9 with a terminal C-C triple bond in 88% yield. Fe(III)-catalyzed aerobic oxidation of 9 afforded aldehyde 10 in 62% yield [46] . Wittig olefination of the aldehyde functionality in 10 afforded the terminal alkyne 1c [47] , which underwent the ATA (allenylation of terminal alkynes) reaction with methyl 4-oxobutanoate 2k (readily available from γ-butyrolactone in 2 steps [48] ) in the presence of diphenylprolinol rac - 3a in a sealed tube at 130 °C [49] to yield 4,5-allenoate rac - 4ck in 64% yield. Through hydrolysis, allenoic acid rac - 5k was prepared in 96% yield with a d.r. 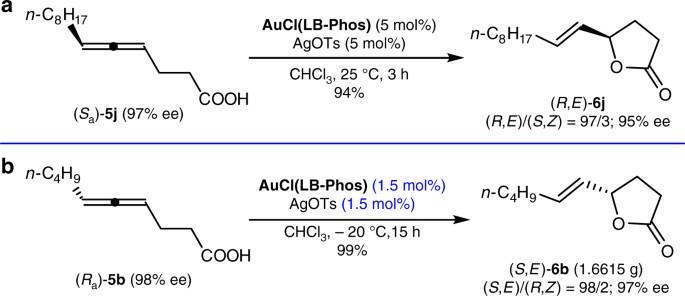Fig. 4 Extended scope of Au-catalyzed cycloisomerization reaction.aSynthesis of the enantiomer (R,E)-butyrolactone6j;bGram scale synthesis for γ-butyrolactone (S,E)-6b of 1.07:1, which underwent the gold-catalyzed cycloisomerization with 10 mol% catalyst at −30 °C for 24 h (for details, see Supplementary Table 4 ) to afford rac -xestospongiene in an excellent yield and E / Z ratio of 99:1 (Fig. 5 ). Fig. 5 First total synthesis of rac -xestospongiene. Reagents and conditions: i. ethynyl-magnesium bromide (1.7 equiv. ), THF, rt, 12.5 h; ii. NaH (1.0 equiv. ), THF, 0 °C, 0.5 h, then rt, 0.5 h; then MeI (1.2 equiv. ), 0 °C, 2 min, then rt, 5 h; then HCl (aq., 3.0 M), 0 °C, then rt, 1.5 h; iii. Fe(NO 3 ) 3 ∙9H 2 O (8 mol%), TEMPO (8 mol%), NaCl (8 mol%), O 2 balloon, DCM, 25 °C, 12.5 h; iv. CBr 4 (1.5 equiv. ), PPh 3 (3.0 equiv. ), DCM, 0 °C, 0.5 h, then 0 °C ~ rt, 1 h; v. rac - 3a (1.5 equiv. ), methyl 4-oxobutanoate 2k (1.5 equiv. ), CuBr 2 (20 mol%), dioxane, 130 °C, 17 h; vi. LiOH∙H 2 O (1.5 equiv. ), EtOH/H 2 O = 1:1, 90 °C, 1.5 h; vii. 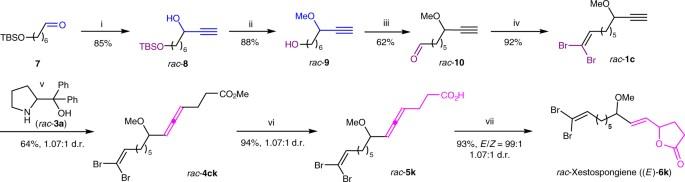Fig. 5 First total synthesis ofrac-xestospongiene. Reagents and conditions: i. ethynyl-magnesium bromide (1.7 equiv.), THF, rt, 12.5 h; ii. NaH (1.0 equiv.), THF, 0 °C, 0.5 h, then rt, 0.5 h; then MeI (1.2 equiv.), 0 °C, 2 min, then rt, 5 h; then HCl (aq., 3.0 M), 0 °C, then rt, 1.5 h; iii. Fe(NO3)3∙9H2O (8 mol%), TEMPO (8 mol%), NaCl (8 mol%), O2balloon, DCM, 25 °C, 12.5 h; iv. CBr4(1.5 equiv.), PPh3(3.0 equiv.), DCM, 0 °C, 0.5 h, then 0 °C ~ rt, 1 h; v.rac-3a(1.5 equiv.), methyl 4-oxobutanoate2k(1.5 equiv.), CuBr2(20 mol%), dioxane, 130 °C, 17 h; vi. LiOH∙H2O (1.5 equiv.), EtOH/H2O = 1:1, 90 °C, 1.5 h; vii. AuCl(LB-Phos) (10 mol%), AgOTs (10 mol%), CHCl3, -30 °C, 24 h AuCl(LB-Phos) (10 mol%), AgOTs (10 mol%), CHCl 3 , -30 °C, 24 h Full size image Asymmetric synthesis of xestospongienes E–H It is well known that different stereoisomers of drug molecules may show very distinct biological activities. After methylation, deprotection, aerobic oxidation, and Wittig olefination reaction, ( R )- 8 and ( S )- 8 (for their syntheses, see Supplementary Tables 5 , 6 and Supplementary Methods [50] ) were easily converted to terminal propargylic methyl ethers ( R )- 1c and ( S )- 1c , respectively (Fig. 6a, b ). Fig. 6 First total synthesis of xestospongienes E–H. a Synthesis of ( R )- 1c ; b Synthesis of ( S )- 1c ; c Total synthesis of xestospongiene F; d Total synthesis of xestospongiene G; e Total synthesis of xestospongiene H; f Total synthesis of xestospongiene E. Reagents and conditions: i. NaH (1.0 equiv. ), THF, 0 °C then rt; then MeI (1.2 equiv. ), 0 °C ~rt; then HCl (aq., 3.0 M), MeOH, rt; ii. Fe(NO 3 ) 3 ∙9H 2 O (10 mol%), TEMPO (10 mol%), NaCl (10 mol%), O 2 balloon, DCM, rt; iii. CBr 4 (1.5 equiv. ), PPh 3 (3.0 equiv. ), DCM, 0 °C; iv. methyl 4-oxobutanoate 2k (1.5–1.7 equiv. ), CuBr 2 (20 mol%), dioxane, 120 °C; v. LiOH∙H 2 O (1.5 equiv. ), EtOH/H 2 O = 1:1, 90 °C; vi. AuCl(LB-Phos) (10 mol%), AgOTs (10 mol%), CHCl 3 , −30 °C Full size image The reaction of ( R )- 1c , 2k , and ( S )-diphenylprolinol ( S )- 3a in a ratio of 1:1.5:1.5 afforded ( R a , R )- 4ck as a single stereoisomer in 47% yield with >99% ee and >99:1 d.r. Hydrolysis of ( R a , R )- 4ck was conducted subsequently by its treatment with LiOH∙H 2 O at 90 °C for 1.5 h affording ( R a , R )- 5k , which was cycloisomerized with 10 mol% of AuCl(LB-Phos) at −30 °C to afford (5 S ,1′ E ,3′ R )- 6k , i.e., xestospongiene F (reported as xestospongiene E [4] ) in 94% yield with >99% ee and >99:1 d.r (Fig. 6c ). Xestospongienes G, H, and (5 R ,1′ E ,3′ S )- 6k , i.e., xestospongiene E (reported as Xestospongiene F [4] ) could also be obtained easily with high stereo- and enantioselectivity in a similar way by just replacing amino alcohol ( S )- 3a with ( R )- 3a or propargylic alcohol ( R )- 1c with ( S )- 1c (Fig. 6d–f ). Subsequently, gram scale synthesis of xestospongiene F was easily realized with a high enantiopurity (99% ee and 98:2 d.r.) (for details, see Supplementary Methods). 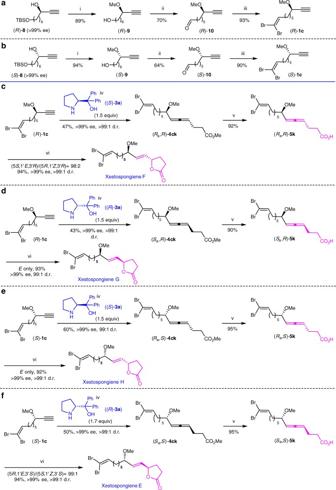Fig. 6 First total synthesis of xestospongienes E–H.aSynthesis of (R)-1c;bSynthesis of (S)-1c;cTotal synthesis of xestospongiene F;dTotal synthesis of xestospongiene G;eTotal synthesis of xestospongiene H;fTotal synthesis of xestospongiene E. Reagents and conditions: i. NaH (1.0 equiv.), THF, 0 °C then rt; then MeI (1.2 equiv.), 0 °C ~rt; then HCl (aq., 3.0 M), MeOH, rt; ii. Fe(NO3)3∙9H2O (10 mol%), TEMPO (10 mol%), NaCl (10 mol%), O2balloon, DCM, rt; iii. CBr4(1.5 equiv.), PPh3(3.0 equiv.), DCM, 0 °C; iv. methyl 4-oxobutanoate2k(1.5–1.7 equiv.), CuBr2(20 mol%), dioxane, 120 °C; v. LiOH∙H2O (1.5 equiv.), EtOH/H2O = 1:1, 90 °C; vi. AuCl(LB-Phos) (10 mol%), AgOTs (10 mol%), CHCl3, −30 °C 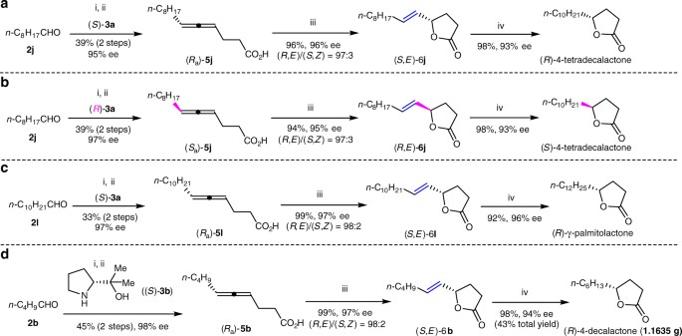Fig. 7 Synthesis of biologically active aliphatic γ-butyrolactones.aSynthesis of biologically active (R)-4-tetradecalactone;bSynthesis of biologically active (S)-4-tetradecalactone;cSynthesis of biologically active (R)-γ-palmitolactone;dSynthesis of biologically active (R)-4-decalactone. Reagents and conditions: i. ethyl pent-4-ynoate1b(1.2 equiv.),2(1.5 equiv.),3(1.0 equiv.), CuBr2(20 mol%), dioxane, 120 °C; ii. LiOH∙H2O (1.5 equiv.), EtOH/H2O = 1:1, 90 °C; iii. AuCl(LB-Phos)/AgOTs (1.5–5 mol%), CHCl3; iv. Pd/C (2.4–5 mol%), H2(25 atm), EtOAc, rt Asymmetric syntheses of naturally occurring γ-alkylic γ-lactones As stated above, aliphatic γ-butyrolactones are the major aroma components of many industrial fragrances and ingredients in flavors and as food additives [11] , some of which also work as quorum-sensing molecules in vivo [51] . Hydrogenation of the C=C bond in ( E )-alkenyl γ-butyrolactones E - I would provide an efficient entry to these naturally occurring γ-alkylic γ-lactones II listed in Fig. 1b , provided that the cleavage of the allylic C–O bond causing racemization to the chiral center under the transition metal catalysis may be avoided. It has been established that the two enantiomers of γ-alkylic γ-butyrolactones made some differences in odor quality and odor intensity [11] , [52] , [53] . Thus, we tried to synthesize both ( R ) and ( S )-γ-lactones by utilizing the current strategy. Starting from asymmetric allenylation of readily available ethyl pent-4-ynoate 1b with nonanal 2j in the presence of ( S )- 3a , followed by hydrolysis, 4,5-allenoic acid ( R a )- 5j was afforded in 39% yield with 95% ee. Subsequent Au-catalyzed cycloisomerization of ( R a )- 5j was executed to yield γ-butyrolactone bearing a trans C=C bond ( S , E )- 6j in 96% yield with 96% ee and 97:3 E / Z . ( R )-4-tetradecalactone was obtained by hydrogenation of ( S , E )- 6j in the presence of 5 mol% Pd/C in 98% yield with 93% ee (Fig. 7a ) [30] , [31] , [54] , [55] . Fig. 7 Synthesis of biologically active aliphatic γ-butyrolactones. a Synthesis of biologically active ( R )-4-tetradecalactone; b Synthesis of biologically active ( S )-4-tetradecalactone; c Synthesis of biologically active ( R )-γ-palmitolactone; d Synthesis of biologically active ( R )-4-decalactone. Reagents and conditions: i. ethyl pent-4-ynoate 1b (1.2 equiv. ), 2 (1.5 equiv. ), 3 (1.0 equiv. ), CuBr 2 (20 mol%), dioxane, 120 °C; ii. LiOH∙H 2 O (1.5 equiv. ), EtOH/H 2 O = 1:1, 90 °C; iii. AuCl(LB-Phos)/AgOTs (1.5–5 mol%), CHCl 3 ; iv. Pd/C (2.4–5 mol%), H 2 (25 atm), EtOAc, rt Full size image The enantiomer ( S )-4-tetradecalactone was executed by following the same synthetic route just by replacing ( S )- 3a with ( R )- 3a in the step of EATA (enantioselectivi allenylation of terminal alkynes) reaction, giving the desired product with a similar yield and enantioselectivity (Fig. 7b ) [30] , [55] . Similarly, naturally occurring aromatic ( R )-γ-palmitolactone was synthesized in 96% ee by just using undecanal 2l as the starting aldehyde in EATA reaction (Fig. 7c ) [56] . ( R )-4-Decalactone is a sex pheromone of Osmoderma eremite released mainly or exclusively by male beetles [57] , which has also proven to be cytotoxic [58] , [59] , and synthesized with biocatalysts [26] , [58] , [59] or by other strategies [29] , [53] , [60] . Gram scale synthesis of ( R )-4-decalactone was also realized easily in 43% total yield for 4 steps with 94% ee (Fig. 7d ). A facile strategy for general asymmetric synthesis of two types of common γ-butyrolactones from readily available common chemicals-terminal alkynes and aldehydes-has been developed by applying the newly identified catalyst, AuCl(LB-Phos), with the stereoselectivity of up to >99:1 E / Z and >99% ee. The first total syntheses of xestospongienes E, F, G, and H have been realized with high stereoselectivity. In addition, the C–O bond cleavage-free hydrogenation led to a general access to naturally occurring γ-alkyl γ-butyrolactones, such as ( R )-4-tetradecalactone, ( S )-4-tetradecalactone, ( R )-γ-palmitolactone, and ( R )-4-decalactone, efficiently with ee of 93–96%. Such a modular solution to two different types of optically active γ-butyrolactones will surely stimulate further interest in the synthetic and bio-potential of these compounds and identifying even better aromas for human life. Further studies on this area are being carried out in our laboratory. General method for cycloisomerization of alkadienoic acids To a dry Schlenk tube were added AgOTs (0.0142 g, 0.05 mmol, weighed in glove box, 98%), AuCl(LB-Phos) (0.0299 g, 0.05 mmol), and CHCl 3 (5 mL) under nitrogen atmosphere sequentially. After stirring for 15 min, ( R )-trideca-4,5-allenoic acid ( R a )- 5a (0.2108 g, 1 mmol) and CHCl 3 (5 mL) were added. After being continuously stirred at 25 °C for 3 h, the reaction was complete as monitored by thin layer chromatography (TLC). Filtration through a short column of silica gel [eluent: Et 2 O (20 mL × 3)] and evaporation afforded a crude mixture of ( S , E )- 6a and ( R , Z )- 6a (( S , E ) / ( R , Z ) = 97:3, as determined by 1 H NMR analysis). Column chromatography on silica gel afforded ( S , E )- 6a (0.2017 g, 96%, ( S , E ) / ( R , Z ) = 98:2 as determined by 1 H NMR analysis) [eluent: petroleum ether (60–90 °C)/ethyl acetate = 15/1 (400 mL) to 10/1 (550 mL)] as an oil with pleasant flavor: 96% ee (HPLC conditions: Chiralcel OJ-H column, n -hexane/ i -PrOH = 200/1, 1.0 mL/min, λ = 214 nm, t R (major) = 22.73 min, t R (minor) = 20.86 min); [ α ] D 20 = + 29.6 ( c = 1.01, CHCl 3 ); 1 H NMR (300 MHz, CDCl 3 ) δ 5.81 (dt, J 1 = 15.3 Hz, J 2 = 7.2 Hz, 1H, =CH), 5.49 (dd, J 1 = 15.3 Hz, J 2 = 7.2 Hz, 1H, =CH), 4.90 (q, J = 7.2 Hz, 1H, CH), 2.61–2.50 (m, 2H, CH 2 ), 2.46–2.31 (m, 1H, one proton from CH 2 ), 2.13–1.90 (m, 3H, CH 2+ one proton from CH 2 ), 1.45–1.18 (m, 10H, CH 2 × 5), 0.88 (t, J = 6.6 Hz, 3H, CH 3 ); the following signals are discernible for ( R , Z )- 6a : δ 5.72–5.62 (m, 1H, =CH), 5.31–5.21 (m, 1H, CH); 13 C NMR (75 MHz, CDCl 3 ) δ 177.0, 135.6, 127.2, 81.1, 32.0, 31.6, 29.0, 28.9, 28.7, 28.64, 28.61, 22.5, 14.0; IR (neat) ν (cm −1 ) 2955, 2926, 2855, 1778, 1673, 1459, 1415, 1378, 1327, 1296, 1216, 1177, 1123, 1010; GC-MS (GC condition: injector: 280 °C; column: DB5 column 30 m × 0.25 mm, temperature programming: 60 °C (2 min), 20 °C/min to 280 °C, 280 °C (30 min); detector: 280 °C) (70 ev, EI) m/z (%) for ( S , E )- 6a : t R (major) = 5.83 min: 210 (M + , 2.31), 111 (100); for ( R , Z )- 6a : t R (minor) = 5.76 min: 210 (M + , 0.75), 111 (100). HRMS calcd for C 13 H 22 O 2 [M + ]: 210.1620, found: 210.1624. Data availability All data that support the findings of this study are available in the online version of this paper in the accompanying Supplementary Methods (including experimental procedures, compound characterization data). The X-ray crystallographic coordinates for structure of AuCl(LB-Phos) reported in this study has been deposited at the Cambridge Crystallographic Data Centre (CCDC), under deposition number CCDC 1558142. This data can be obtained free of charge from The Cambridge Crystallographic Data Centre via www.ccdc.cam.ac.uk/data_request/cif .